Mapping the evolution of hierarchical microstructures in a Ni-based superalloy Phase separation of γ′ precipitates determines the microstructure and mechanical properties of nickel-based superalloys. In the course of ageing, disordered γ spheres form inside ordered (L1 2 ) γ′ precipitates, undergo a morphological change to plates and finally split the γ′ precipitates. The presence of γ particles inside γ′ affects coarsening kinetics and increases alloy hardness. Here we use atom probe tomography to visualize phase separation in a Ni 86.1 Al 8.5 Ti 5.4 alloy in three dimensions and to quantify the composition of all the phases with near-atomic resolution. We find that γ′ precipitates are supersaturated in nickel, thereby driving the formation of γ particles and observe a compositional evolution of the γ particles, which accompanies their morphological change. Our results suggest that by controlling nickel supersaturation we can tailor the phase separation and thereby the properties of nickel-based superalloys. Phase-separation phenomena occur in a variety of alloys and their understanding is of essential importance for modern alloy design. In superalloy metallurgy, Ni-Al-Ti is one of the most important alloy systems [1] showing a typical γ/γ′ two-phase microstructure. A particular phase-separation phenomenon, namely, the formation of further particles inside γ′ precipitates, has captured the attention of researchers. Although first observed in the 1960s when a fine dispersion of unknown particles inside the γ′ precipitates of a Ni-based alloy was reported [2] , it took another 10 years to suggest the particles (in Udimet 700) to be a carbide of perovskite type [3] . Shortly after, it was alternatively proposed that the particles (in IN-738) may be γ phase [4] , [5] . Later, it was claimed that these γ particles suppress the coarsening of the γ′ precipitates of a Ni-Al-Ti alloy on ageing and finally induce a split of the γ′ precipitates and thus refine the microstructure [6] . This behaviour is not only fascinating from the scientific point of view but also technologically important because of the associated potential to strengthen alloys. Other alloy systems [7] , [8] , [9] have also been reported to exhibit similar phase-separation phenomena. In so-called ‘inverse’ alloys, γ′ can serve as a matrix for γ precipitates [10] , [11] , [12] , [13] that act in a similar way as γ particles inside γ′ precipitates [6] . The three-dimensional (3D) morphology and spatial distribution of γ plates inside γ′ precipitates of a Ni-Al-Ti alloy has been studied by transmission electron tomography [14] . Attempts have been made to identify such γ particles and measure their chemical composition using electron energy loss spectroscopy and energy dispersive X-ray spectroscopy (EDS). Owing to the limited spatial and analytical resolution of these methods, only the ratio of Ti contents between the γ′ precipitates and the γ particles has been determined but not their composition [14] . Recently, during the early stages of decomposition of γ′ precipitates of a Ni-Al-Ti alloy, the formation of Ni-rich clusters has been shown by statistical analysis of atom probe tomography (APT) data [15] . However, even these advanced analytical studies did not reveal the chemical nature of the nanometre-scaled γ particles. Laser-assisted wide-angle APT, which has been significantly developed over the past decade [16] , allows for a 3D site-specific analysis of heterogeneities with sizes from a few atoms to 200 nm in volumes of up to 10 8 nm 3 with near-atomic resolution at high detection rates [17] . Here we elucidate microstructural and chemical features of phase separation in γ′ precipitates in a Ni-Al-Ti model alloy combining transmission electron microscopy (TEM) and laser-assisted wide-angle APT. In this alloy, phase separation is introduced by subsequent ageing during which γ particles form inside γ′ precipitates. We find that the coalescence of Ni-rich clusters leads to the formation of γ particles during ageing at 1,023 ϰ. These γ particles hinder the growth of γ′ precipitates and limit their size. Furthermore, the presence of γ particles inside γ′ precipitates increases the overall alloy hardness. By means of alloy design and thermal treatment, the amount of Ni-supersaturation of γ′ precipitates could be controlled to tailor the microstructure and mechanical properties of Ni-based superalloys. 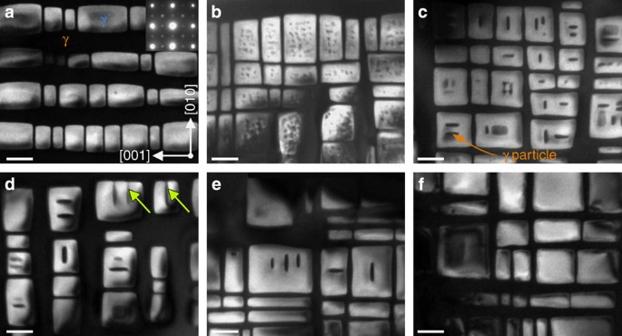Figure 1: DF-TEM images before and after phase separation. (a) Ordered (L12) γ′ precipitates in a disordered (A1) γ matrix after homogenizing Ni86.1Al8.5Ti5.4at 1,548 K/4 h and ageing at 1,213 K for 0.75 h. The selected area electron diffraction pattern in the inset represents field of view ofa. (b) γ spheres form when subsequently aged at 1,023 K for 6 h. (c) The γ spheres undergo a morphological transformation to plates after further ageing for 24 h. (d) The γ plates split the γ′ precipitates (indicated by arrows) when further aged for 96 h. (e,f) After split of γ′ precipitates, γ plates merge with the γ matrix after ageing for 192 and 384 h, respectively. Phase-separated microstructure Figure 1a shows a dark-field (DF) TEM image and the corresponding selected area electron diffraction pattern of a Ni 86.1 Al 8.5 Ti 5.4 alloy after homogenization at 1,548 K for 4 h and ageing at 1,213 K for 0.75 h. We observe a microstructure consisting of cuboid γ′ precipitates embedded in the γ matrix. The [001] zone axis diffraction pattern in the inset of Fig. 1a clearly reveals superlattice reflections of the L1 2 crystal structure (Cu 3 Au type), which derive from ordered γ′ precipitates. The γ′ precipitates are aligned along the <001>γ matrix directions. Since the γ′ precipitates were imaged by a (110) superlattice reflection they appear bright, whereas dark regions correspond to the disordered (A1) γ matrix (γ m ). Subsequent ageing at 1,023 K leads to secondary phase separation during which disordered γ particles (γ p , dark) form inside the γ′ precipitates (γ′) thus building a hierarchical microstructure γ m ⊃ γ′ ⊃ γ p ( Fig. 1b–f ). After 6 h of ageing, γ particles appear as spheres inside the γ′ precipitates and are accompanied by a particle-free zone at the γ′ periphery ( Fig. 1b ). When aged for 24 h, the γ spheres coalesce and change their shape from spheres to plates ( Fig. 1c ). After ageing for 96 h some of the γ plates reach the γ′ interface and eventually split the γ′ precipitates (indicated by arrows in Fig. 1d ). In the course of further ageing for 192 and 384 h ( Fig. 1e,f ), the γ plates grow and the smaller γ′ precipitates no longer contain γ plates since these have merged with the surrounding γ matrix after splitting the γ′ precipitates. Figure 1: DF-TEM images before and after phase separation. ( a ) Ordered (L1 2 ) γ′ precipitates in a disordered (A1) γ matrix after homogenizing Ni 86.1 Al 8.5 Ti 5.4 at 1,548 K/4 h and ageing at 1,213 K for 0.75 h. The selected area electron diffraction pattern in the inset represents field of view of a . ( b ) γ spheres form when subsequently aged at 1,023 K for 6 h. ( c ) The γ spheres undergo a morphological transformation to plates after further ageing for 24 h. ( d ) The γ plates split the γ′ precipitates (indicated by arrows) when further aged for 96 h. ( e , f ) After split of γ′ precipitates, γ plates merge with the γ matrix after ageing for 192 and 384 h, respectively. Full size image To compare size of γ′ precipitates and γ particles of different shapes, their equivalent radius was considered, defined as R =( A /π) 0.5 , where A=a × b is the area of a γ′ precipitate or a γ particle determined by measuring the perpendicular sides a and b (with a≥b ). The average equivalent radius <R> is given by the mean of 100 γ′ precipitates and up to 1,000 γ particles for each state. 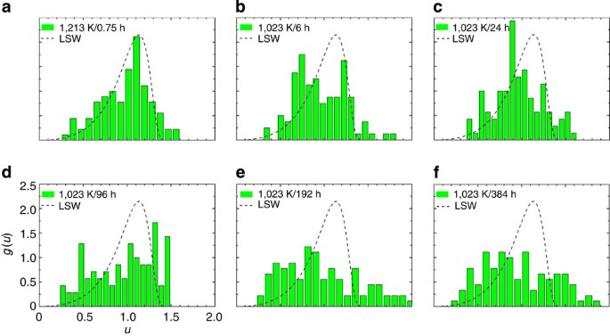Figure 2: PSDs for γ′ precipitates. The scaled PSDs for γ′ are compared with the prediction of the LSW coarsening theory by Lifshitz and Slyozov18and Wagner19(dashed line). The probability density isg(u)andu=R/<R>is the scaled particle radius, whereRis the equivalent radius of a γ′ precipitate and<R>is the average equivalent radius of 100 γ′ precipitates. This is shown after ageing at (a) 1,548 K/4 h+1,213 K/0.75 h and subsequently at 1,023 K for (b) 6 h, (c) 24 h, (d) 96 h, (e) 192 h and (f) 384 h. Figure 2a–f illustrate the γ′ particle size distribution (PSD) of all the states displayed in Fig. 1a–f . The theoretical Lifshitz–Slyozov–Wagner (LSW) distribution [18] , [19] g(u) , where the normalized radius u is defined as u=R/<R> , is superimposed in Fig. 2a–f . Only for the sample homogenized at 1,548 K for 4 h and aged at 1,213 K for 0.75 h ( Fig. 2a ), the experimentally obtained PSD follows the theoretically predicted distribution, whereas for further ageing ( Fig. 2b–f ) there are large deviations. Figure 2: PSDs for γ′ precipitates. The scaled PSDs for γ′ are compared with the prediction of the LSW coarsening theory by Lifshitz and Slyozov [18] and Wagner [19] (dashed line). The probability density is g(u) and u = R / <R> is the scaled particle radius, where R is the equivalent radius of a γ′ precipitate and <R> is the average equivalent radius of 100 γ′ precipitates. This is shown after ageing at ( a ) 1,548 K/4 h+1,213 K/0.75 h and subsequently at 1,023 K for ( b ) 6 h, ( c ) 24 h, ( d ) 96 h, ( e ) 192 h and ( f ) 384 h. Full size image The number density N v of γ particles inside γ′ precipitates was estimated by counting the number ( N Par ) of such particles shown in TEM images with a foil thickness of ~70 nm. We represent the surface S P of the different particles either by spheres of radius R or by cuboids a=c depending on their shape. Combining the information on mean particle surface and number density, we obtain the specific surface area of γ particles per unit volume as S V =S P × N v . The data are listed in the first two columns of Table 1 . Table 1 Quantities determined by TEM and APT. 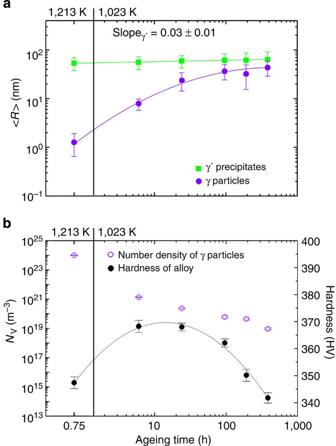Figure 3: Evolution of microstructure and mechanical quantities during ageing. (a) Average equivalent radius<R>of both γ′ precipitates and γ particles in Ni86.1Al8.5Ti5.4. (b) Number densityNVof γ particles and HV of the alloy. The errors are s.d.σand calculated based on counting statistics and s.e. propagation methods31. Full size table Figure 3 demonstrates the course of Vickers hardness (HV), representative of the strength of the alloy, during ageing corresponding to the states shown in Fig. 1a–f . We observe a peak hardness for the samples aged at 1,023 K for 6 and 24 h, after which in the course of further ageing at 1,023 K the hardness decreases. Figure 3: Evolution of microstructure and mechanical quantities during ageing. ( a ) Average equivalent radius <R> of both γ′ precipitates and γ particles in Ni 86.1 Al 8.5 Ti 5.4 . ( b ) Number density N V of γ particles and HV of the alloy. The errors are s.d. σ and calculated based on counting statistics and s.e. propagation methods [31] . Full size image Chemical evolution during phase separation To investigate the chemical origin and the temporal evolution of phase separation in γ′ precipitates, we performed APT analyses on samples representing three different states: before phase separation ( Fig. 1a ), an early stage characterized by the presence of γ spheres ( Fig. 1b ) and a later stage with γ plates ( Fig. 1c ). The analyses of the samples shown in Fig. 1b,c will be visualized. 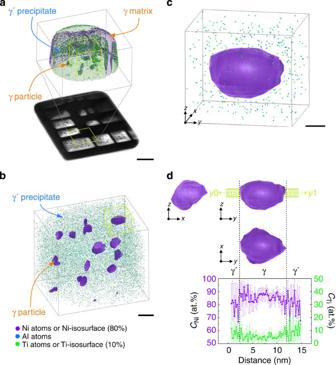Figure 4: Correlation between an APT analysis and DF-TEM image. The image shows a sample after homogenizing Ni86.1Al8.5Ti5.4at 1,548 h/4 h, ageing at 1,213 K/0.75 h and subsequently at 1,023 K/6 h. (a) The APT volume where γ spheres (purple) can be seen inside the γ′ precipitates, represented by 80 at.% Ni or 10 at.% Ti iso-concentration surfaces, respectively, corresponds to the yellow box in the DF-TEM image. (b) A further magnified region is shown, which corresponds to the yellow box in the APT volume ofa. (c,d) Detailed analysis of the individual γ sphere marked by a yellow box inb. (d) Different projections and a concentration profile for Ni and Ti (at.%) are shown. The errors are s.d., 2σ. Scale bar, 100 nm (a); 10 nm (b); and 2 nm (c) (widths). Figure 4a correlates an atom probe tomogram image and a DF-TEM of the sample aged at 1,023 K for 6 h (same state as in Fig. 1b ). The DF-TEM image was tilted into the x – y plane to match the APT presentation. The APT reconstruction shown in Fig. 4a corresponds to the region indicated by a rectangle in the DF-TEM image (with further magnification shown in Fig. 4b ). For the sake of clarity, only one-third of the entire APT data set is shown, corresponding to a volume of 130 × 130 × 75 nm 3 . Both γ matrix and the γ spheres are visualized by an 80 at.% Ni iso-concentration surface (purple). The γ′ precipitates are represented using a 10 at.% Ti iso-concentration surface (green) since Ti is a γ′-forming element [14] . To reveal the γ spheres inside the γ′ precipitate, the iso-concentration surfaces are made translucent. An enlarged presentation of a sub-volume of 50 × 60 × 50 nm 3 of the γ′ precipitate in the foreground is separated to highlight the morphology and the spatial distribution of the γ spheres ( Fig. 4b ). In this image area, γ spheres are displayed by a closed iso-concentration surface (purple). For a clear visualization of the γ spheres, only 2% of the measured Al and Ti atoms in the surrounding are shown by the visualization software. The interior of the selected γ′ precipitate comprises ~15 γ spheres with radii from 2 to 8 nm, of which only two deviate from ideal spherical geometry and appear as interconnected particles. The average radius of the γ spheres is 6 nm. Figure 4c illustrates a single γ sphere labelled by a yellow box in Fig. 4b . This γ sphere was further investigated and is shown in Fig. 4d in x – z , y – z and y – x projections. In the z – y projection, the γ sphere appears slightly compressed along the z axis. The concentration profile from y 0 to y 1 along the yellow cylinder ( r =1 nm) was calculated for Ni and Ti, and is shown in Fig. 4d . In this concentration profile, each point averages ~100 atoms (corresponding to a few atomic planes within the truncated cylinder), resulting in a relatively large s.d., σ . The s.d., σ for the elemental concentration C i is given by ( C i (1− C i )/ N ) 0.5 , where N is the total number of atoms in the analysed volume. The dashed lines indicate interfaces between the γ sphere and the γ′ precipitate. The average compositions of the γ matrix, γ′ precipitates and γ spheres as derived from APT analysis are given in Table 2 . The volume fraction ϕ γ′ of γ′ precipitates is calculated based on the lever rule approach [20] , the composition of γ′ precipitates from Table 2 and is given in Table 1 . Figure 4: Correlation between an APT analysis and DF-TEM image. The image shows a sample after homogenizing Ni 86.1 Al 8.5 Ti 5.4 at 1,548 h/4 h, ageing at 1,213 K/0.75 h and subsequently at 1,023 K/6 h. ( a ) The APT volume where γ spheres (purple) can be seen inside the γ′ precipitates, represented by 80 at.% Ni or 10 at.% Ti iso-concentration surfaces, respectively, corresponds to the yellow box in the DF-TEM image. ( b ) A further magnified region is shown, which corresponds to the yellow box in the APT volume of a . ( c , d ) Detailed analysis of the individual γ sphere marked by a yellow box in b . ( d ) Different projections and a concentration profile for Ni and Ti (at.%) are shown. The errors are s.d., 2 σ . Scale bar, 100 nm ( a ); 10 nm ( b ); and 2 nm ( c ) (widths). Full size image Table 2 Chemical compositions (at.%) of all phases in Ni 86.1 Al 8.5 Ti 5.4 . 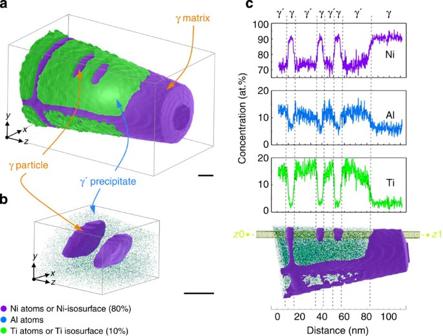Figure 5: APT analysis revealing γ plates in a γ′ precipitate. Here the analysis of a sample of Ni86.1Al8.5Ti5.4after homogenization at 1,548 K/4 h, ageing at 1,213 K/0.75 h and subsequently at 1,023 K/24 h is shown. (a) The iso-concentration surface exhibits four truncated γ′ precipitates (green). The top front one contains two γ plates. (b) These are extracted for a detailed view. (c) Concentration profiles for Ni, Al and Ti, clearly revealing the alternating phases. Scale bar, 10 nm (widths). Full size table Figure 5a displays a 3D reconstruction of an APT analysis of a sample aged at 1,023 K for 24 h (same state as in Fig. 1c ). In the volume of 55 × 55 × 120 nm 3 , we observe four truncated γ′ precipitates (green) embedded in the γ matrix (purple). The γ′ precipitate at the top front contains two truncated γ plates (purple). The morphology of these γ plates is illustrated in Fig. 5b . If one-third of the full γ′ precipitate was captured by APT (this seems likely in view of the TEM images), the mean radius of the γ′ precipitate would be 28 nm, whereas the average thickness of both γ plates would be about 8 nm and the radius ~9 nm. The distance between the γ plates is 9 nm with a distance to the γ′ precipitate edges of 20 nm. These findings are in agreement with TEM observations ( Fig. 1c ). Figure 5c gives the concentration profiles along a cylinder from z 0 to z 1 positioned perpendicular to the γ/γ′ interfaces as indicated in Fig. 5c . The course of the concentrations of Ni, Al and Ti clearly indicates alternating phases, namely, γ′ precipitate, γ matrix, γ′ precipitate, γ plate, γ′ precipitate, γ plate, γ′ precipitate and γ matrix. The results of a detailed APT analysis of the composition of the γ matrix, γ′ precipitates and γ plates are listed in Table 2 . Figure 5: APT analysis revealing γ plates in a γ′ precipitate. Here the analysis of a sample of Ni 86.1 Al 8.5 Ti 5.4 after homogenization at 1,548 K/4 h, ageing at 1,213 K/0.75 h and subsequently at 1,023 K/24 h is shown. ( a ) The iso-concentration surface exhibits four truncated γ′ precipitates (green). The top front one contains two γ plates. ( b ) These are extracted for a detailed view. ( c ) Concentration profiles for Ni, Al and Ti, clearly revealing the alternating phases. Scale bar, 10 nm (widths). Full size image On the basis of quantities derived from TEM and APT analyses, for example, the specific surface S V of γ particles and the molar volume V m of γ′ precipitates given by V m =Σ( V i × C i ), we can calculate the molar surface energy E m of γ particles as E m = S V × V m × γ S . Therefore, V i is the molar volume of the pure element i and C i is its concentration in the γ′ precipitate with γ S the surface energy density (γ S =0.018 J m −2 ) [6] . When calculating V m for all ageing times, we assume that the composition of γ′ precipitates does not change during ageing at 1,023 K for 24–384 h. Furthermore, using the composition of γ′ precipitates given in Table 2 and mixing enthalpies of three binary subsystems [21] , we obtain the molar Gibbs free energy G mix of γ′ precipitates also listed in Table 1 . Using TEM and APT analyses, we have clarified the chemical identity of nanometre-scaled γ particles (enriched in Ni) to elucidate the origin and the evolution of phase separation in a Ni-based model superalloy. As demonstrated in a previous study [15] , APT analysis reveals nanometre-sized Ni-rich clusters inside the γ′ precipitates of samples showing a typical γ+γ′ two-phase microstructure in an early stage comparable to Fig. 1a . We also found Ni-rich clusters inside γ′ precipitates in samples after homogenization at 1,548 K for 4 h and ageing at 1,213 K for 0.75 h by statistical analysis of APT data (not shown here). Coalescence of Ni-rich clusters gives rise to the formation of γ spheres, which evolve to equilibrium γ phase, accompanied by a morphological transformation from spheres to plates. This morphological transformation (from Fig. 1b to c ) is driven by the relative gain of elastic energy to interfacial energy, which increases with particle size [6] , [22] , [23] . The γ plates become aligned along the elastically soft <001> directions [22] of the γ′ precipitates, which is energetically favourable because of the elastic interaction between the particles [6] . The LSW theory predicts coarsening of γ′ with time, t , according to R 3 −R 0 3 =kt , where R 0 is the average radius at the onset of coarsening and k is a volume fraction-dependent rate constant. According to LSW theory, the predicted radius evolution can be approximated by a R t 0.33 relation, whereas in this study we observe R t 0.03 ± 0.01 , which suggests that coarsening of γ′ precipitates is largely suppressed during formation and growth of γ particles ( Fig. 3a ), which has also been reported elsewhere [6] . Further growth of γ plates splits γ′ precipitates ( Fig. 1d–f ), which was suggested to refine the γ/γ′ microstructure [6] . This would be highly desirable in terms of thermo-mechanical properties and stability of alloys such as Ni-based superalloys that are hardened by precipitates. However, after splitting of γ′ precipitates, we find that the PSDs ( Fig. 2a–f ) reveal a broadening and significant deviations from the LSW theory [18] , [19] . In addition, the peak hardness in Fig. 3b is correlated with the presence of γ spheres and γ plates at ageing times of 6 and 24 h, respectively, and not with the later stages. Moreover, the number density N V of γ particles ( Fig. 3b ) decreases on further ageing during which splitting of γ′ precipitates takes place. Appreciable hardening of ordered γ′ phase was attributed to precipitation of γ in an ‘inverse’ alloy (γ′ matrix) [24] , since γ in γ′ increases shearing resistance of γ′ and therefore increases the overall hardness of the alloy. Thus, accounting for the hardening of γ′ precipitates [25] , it is more desirable to retain γ particles inside the γ′ precipitates rather than to provoke their split. An enhanced fraction of γ particles can be achieved by increasing the γ′ volume fraction ϕ γ′ and their size. Thus, we expect the hardening effect to be stronger at higher ϕ γ′ . In previous studies, only microstructural (two-dimensional) and morphological (3D) features of γ particles in γ′ precipitates have been reported [6] , [14] but no entire chemical quantities. Here we find that the amount of Ni in γ′ precipitates in the sample after homogenization at 1,548 K for 4 h and ageing at 1,213 K for 0.75 h is higher (>2 at.%) than the stoichiometric composition of γ′ precipitates. Hence, Ni-supersaturation is the initial driving force for phase separation of γ′ precipitates. Although large surface, and therefore molar surface energy E m , are created, Ni-supersaturation promotes the formation of Ni-rich clusters [15] since this locally decreases the molar Gibbs free energy ( Table 1 ). Subsequently, the large surface energy will be reduced by coalescence of clusters, which results in the formation of γ spheres when aged at 1,023 K for 6 h. These γ spheres lie within the γ+γ′ two-phase region of the ternary phase diagram of Ni-Al-Ti at 1,023 K [26] and are thermodynamically metastable, which still provides a driving force for further phase separation. After a morphological change from initially spheres to plates, the γ plates inside γ′ achieve the equilibrium composition of the γ phase ( Table 2 ). Selective elemental mapping using electron energy loss spectroscopy (Ti-L 2,3 ionization edges) with a spatial resolution below 100 nm recently revealed that contents of Ti in the γ′ precipitates and in the γ particles show a ratio of 2:1–3:1 for a sample aged at 1,023 K for 48 h (ref. 14 ). Contrary to these findings, we observe a ratio of 2:1 for the 6 h and 4:1 for the 24 h aged samples. The composition of the γ matrix was determined as Ni 91 Al 6 Ti 3 by EDS, which is in excellent agreement with our results for the sample aged for 24 h. However, owing to the presence of both γ′ precipitates and γ particles in a typical volume probed by EDS, the measured composition values represent both phases unlike our APT analyses that precisely give the composition of each individual phase. The importance of modern APT for the metallurgist as an analytical technique for the design of advanced materials is apparent. Whether the γ particles will have a beneficial effect on the thermo-mechanical properties and in particular on the morphological change of γ′ precipitates during creep deformation and how to adapt this concept to the more complex commercial usable alloys will have to be shown in the future. Specimen preparation A single-crystal (SX) Ni-based superalloy with a nominal composition of Ni 86.1 Al 8.5 Ti 5.4 (at.%) was cast in a Bridgman furnace [27] , [28] at the University of Bayreuth. The orientation of the SX bar was determined by Laue back reflection to be within 5° of a <001> direction. Discs of 1.5 mm thickness were homogenized at 1,548 K for 4 h to remove dendritic segregation and uniformly disperse the γ′ precipitates in the γ matrix [29] . The homogenized samples were first aged at 1,213 K for 0.75 h and subsequently at 1,023 K for 6, 24, 96, 192 and 384 h. All samples were heat treated in a quenching furnace under flowing argon. Each heat treatment was followed by quenching in iced water. For TEM investigations, discs of 3 mm diameter were punched out of the aged samples. Thin foils suitable for TEM were prepared by electrolytic jet polishing [15] . For APT analyses, square rods of 0.25 × 0.25 × 15 mm 3 were cut out of the samples. The axis of the rods was parallel to the [001] zone axis. Needle-shaped tips with a radius <50 nm were prepared by electropolishing [15] , [17] . Dark-field transmission electron microscopy For DF-TEM, a Philips CM30 microscope operating at 300 kV and equipped with a LaB 6 cathode was used. The (110) superlattice reflection was used for DF-TEM imaging. The orientation of the foils was tilted to an angle of about 2° relative to the [001] zone axis to ensure best imaging conditions. HV measurements Hardness was measured using a HV indenter with 1.96 N force and 20 s loading time. 3D laser-assisted wide angle APT APT analyses were performed in a local electrode APT built at the University of Münster [30] . Thermally induced field evaporation was performed with fs pulses from a ultraviolet laser ( λ =343 nm, 200 kHz, 30 nJ pulse −1 ). The experimental parameters were set to maintain a detection rate of 0.02–0.04 ions per pulse. For all the measurements, the temperature of the tip was kept at 46 K, the ambient pressure to <10 −8 Pa. Iso-concentration surfaces representing the γ matrix and the γ particles were visualized using a threshold of 80 at.% for Ni. The γ′ precipitates are represented by a 10 at.% Ti iso-concentration surface. The threshold values for iso-concentration surfaces were empirically determined. In all the reconstructions, only 2% of the measured atoms are displayed for the sake of clarity. How to cite this article: Vogel, F. et al. Mapping the evolution of hierarchical microstructures in a Ni-based superalloy. Nat. Commun. 4:2955 doi: 10.1038/ncomms3955 (2013).